Selective fishing induces density-dependent growth Over the last decades, views on fisheries management have oscillated between alarm and trust in management progress. The predominant policy for remedying the world fishing crisis aims at maximum sustainable yield (MSY) by adjusting gear selectivity and fishing effort. Here we report a case study on how striving for higher yields from the Eastern Baltic cod stock by increasing selectivity has become exceedingly detrimental for its productivity. Although there is a successive increase in numbers of undersized fish, growth potential is severely reduced, and fishing mortality in fishable size has increased. Once density-dependent growth is introduced, the process is self-enforcing as long as the recruitment remains stable. Our findings suggest that policies focusing on maximum yield while targeting greater sizes are risky and should instead prioritize catch rates over yield. Disregarding the underlying population structure may jeopardize stock productivity, with dire consequences for the fishing industry and ecosystem structure and function. After a long period of detrimental levels of fishing mortality worldwide [1] , management efforts have contributed to some encouraging signs of fish stock recovery, viz. improved abundance and productivity [2] . One such example is that of the Baltic cod fishery ( Fig. 1 ); after more than two decades of high fishing pressure [3] , the Eastern Baltic cod stock is by commonly used metrics considered recovered [4] , [5] . Exploitation rates have dropped to unexpectedly low levels, and as a result the fishery has since 2011 been Marine Stewardship Council-certified ( www.msc.org ). Preceding the recovery, fishing gear selectivity was improved by gradually increasing mesh size over the past 15 years, thereby also lowering juvenile mortality [6] ; in fact, higher selectivity in the trawl fishery, which dominates the cod fishing industry, has been one of the prime management objectives since the early 1990s (ref. 7 ). There are even ongoing discussions on the benefits of targeting even larger size fish, that is fishing at sizes corresponding to global maximum sustainable yield (MSY) [8] , [9] ; these models have, however, been proved to be based on erroneous assumptions [10] . 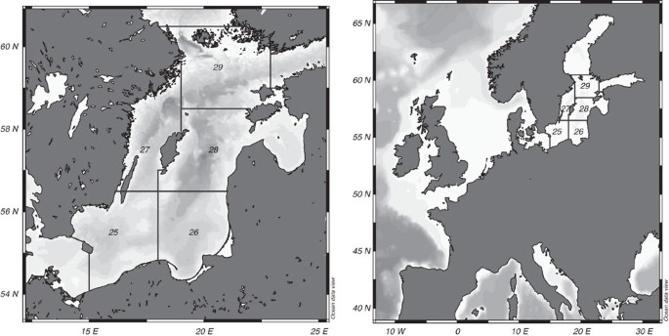Figure 1: The Baltic Sea (left panel) and Europe (right panel). The borders and numbers of the ICES subdivisions are as defined by the International Council for the Exploration of the Sea (www.ices.dk). In recent years, fishing for Eastern Baltic cod takes place almost exclusively in subdivision 25 and 26. Figure 1: The Baltic Sea (left panel) and Europe (right panel). The borders and numbers of the ICES subdivisions are as defined by the International Council for the Exploration of the Sea ( www.ices.dk ). In recent years, fishing for Eastern Baltic cod takes place almost exclusively in subdivision 25 and 26. Full size image Contesting the alleged recovery of the cod stock is the observation that at present the most probable catch in the Baltic consists of malnourished cod at ~38–40 cm (refs 11 , 12 ). The cod fishing industry is faced with dire economic consequences based on the following figures from a fish processing factory unit: between 2006 and 2011, mean landing size declined by 30%, processing time needed increased on a similar scale and filleting yield declined from 36% to 30% ( Fig. 2 ). The poor growth in Eastern Baltic cod has been explained by density dependence resulting from the high average recruitment in recent years [11] . This could be due to either increased interspecific or intraspecific food competition [12] , [13] , [14] , potentially exacerbated by oxygen deficit in bottom water layers [15] . 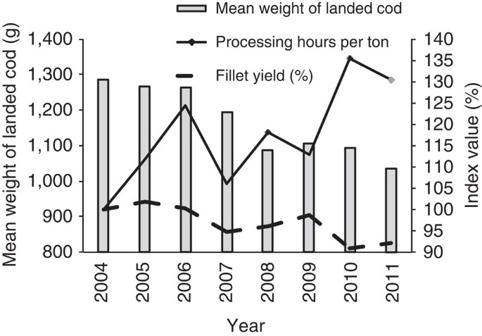Figure 2: Changes in economic variables since 2004. Mean weight of cod landed in the smallest size category (1–2 kg; bars) and yield, that is, fillet obtained from fresh fish combined for all size categories, not including rejected fish (changes in percentage; dashed line), have decreased, whereas processing time per ton of cod has increased (changes in percentages; black line). Figure 2: Changes in economic variables since 2004. Mean weight of cod landed in the smallest size category (1–2 kg; bars) and yield, that is, fillet obtained from fresh fish combined for all size categories, not including rejected fish (changes in percentage; dashed line), have decreased, whereas processing time per ton of cod has increased (changes in percentages; black line). Full size image In this study we assessed growth by applying the von Bertalanffy growth model [16] to fishery-independent data on length at age to depict and analyse changes in population growth. In this growth model, the length (or weight) asymptote of a fish stock, L ∞ , reflects the growth potential of the stock and can be expressed as the predicted mean maximum individual size of a population or cohort. L ∞ varies with feeding conditions, while the catabolic growth coefficient, K , reflects temperature dependence. Incidence of density-dependent growth in combination with management actions intended to increase selectivity towards bigger size classes was early on predicted to be a potentially malicious combination, which may give considerably lower yields than anticipated [16] . Raising length at first catch ( L c ), measured as the 50% point of the selectivity ogive (that is, the curve of a cumulative distribution function), results in increases in intraspecific competition in size groups left unexploited as population density becomes higher, and, consequently, in decreases in L ∞ , that is, in the growth potential of the stock. Lower growth potential at sustained levels of recruitment also leads to crowding, as the number of fish will inevitably increase in non-fishable size groups as growth drops. Consequently, fewer fish will reach fishable sizes—further increases in selectivity might even result in an L c above L ∞ , which means few fish will reach fishable size. Density dependence growth is a prime factor regulating population dynamics [17] , [18] , [19] ; its occurrence after recruitment in exploited fish stocks is a common phenomenon that needs to be considered [20] . Increased population densities may lead to higher natural mortality and lower growth, manifesting as lower L ∞ , seen, for example, in North Sea plaice ( Pleuronectes platessa ) and haddock ( Melanogrammus aeglefinus ) stocks after they had augmented during the period of reduced fishing effort during World War II (ref. 16 ). By contrast, MSY represents a static view on population dynamics; although stock-recruitment relationships are regularly taken into account, density dependence is virtually ignored, while a lower L ∞ inevitably leads to lower MSY. Thus, far from being a conservative approach, MSY-oriented management strategies are focused on ensuring that no potential yield is left unexploited. As a large proportion of all commercial fish stocks have become fully utilized or even depleted over the last decades [1] , density-dependent growth has so far been absent from most management considerations. However, with exploitation rates being adjusted downwards in many parts of the world [2] , and stock recoveries becoming increasingly commonplace, density-dependent growth is likely to be a much more widespread phenomenon, especially in cases where increased selectivity constitutes a vital part of envisaged exploitation patterns [7] , [21] . A more critical investigation of the ecological implications of the MSY concept is therefore needed, including a search for ‘improved’ selectivity in policy making. In this study, we found that increased selectivity in the Eastern Baltic cod fishery leads to higher abundance in non-fishable size groups, leading in turn to lower individual growth. With new recruits entering the population, the lower growth induces crowding in smaller, non-fishable size groups, further decreasing growth potential. Meanwhile, as fishing mortality increases in larger fish groups, the rate of culling by cannibalism between size groups can be expected to be reduced, further aggravating the situation. We reproduce these findings by a model using real estimates on recruitment, L ∞ , mortality rates and selectivity. We argue that the link between higher selectivity and induction of individual density-dependent growth may have implications on MSY-based approaches, in particular when increased selection on larger size classes is an important part of the management strategy. Here we show that the strive for the theoretically highest yields [22] by increasing selectivity is a risk-prone strategy [16] ; as density-dependent growth is induced, stock productivity and population structure may go astray. In search for more robust fisheries management strategies, we argue that catch rates should be prioritized over yield, as it will stabilize yield levels and reduce the need of fishing effort, which will be beneficial for higher ecosystem functionality [13] . Effects of selectivity on growth and population number By exploring existing survey data (see ‘Methods’) we show that L ∞ has radically decreased for cod year classes recruited since 1995, that is, during the period of increased selectivity ( Fig. 3 ). We also found that the catch-per-unit-effort (CPUE) below minimum landing size (MLS), <37 cm, has strongly increased since the year 2000 ( Fig. 4 ). However, after a period of substantially reduced fishing effort during 2007–2008, with a corresponding notable increase in CPUE above MLS, the CPUE in all fishable sizes dropped conspicuously. This downturn in CPUE was even more dramatic for sizes >45 cm in length; in other words, almost no fish above the present L ∞ have been caught in recent years. 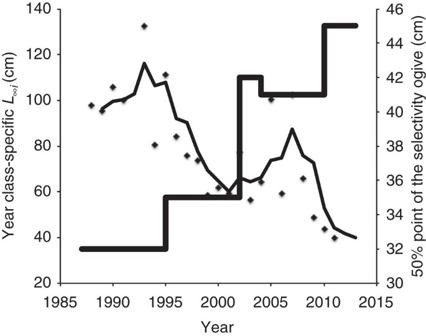Figure 3: The 50% point of the selectivity ogive versus growth potential,L∞i, in Eastern Baltic cod. The prevailing 50% point of the trawl selectivity ogive,Lc, over time is indicated by a black bar (back-shifted 2 years so as to correspond to year classes at age 2 years). Mean asymptotic length,L∞i, for year class,i, mirroring growth potential (black rhomboids), has dropped conspicuously since 1995 (shown by a 3-year moving average). Correlation betweenLcandL∞i, Spearman’sρ=−0.66 (P<0.001). Figure 3: The 50% point of the selectivity ogive versus growth potential, L ∞ i , in Eastern Baltic cod. The prevailing 50% point of the trawl selectivity ogive, L c , over time is indicated by a black bar (back-shifted 2 years so as to correspond to year classes at age 2 years). Mean asymptotic length, L ∞ i , for year class, i , mirroring growth potential (black rhomboids), has dropped conspicuously since 1995 (shown by a 3-year moving average). Correlation between L c and L ∞ i , Spearman’s ρ =−0.66 ( P <0.001). 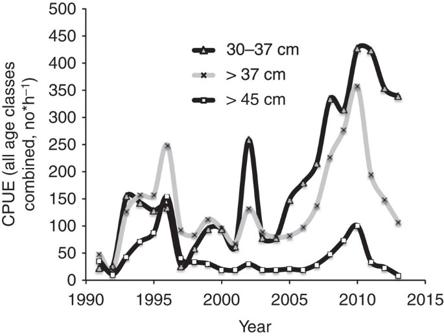Figure 4: Mean annual catch per unit effort (CPUE) for Eastern Baltic cod. The CPUE for the size group 30–37 cm (black line with triangles) has dramatically increased since the millennium shift, while the CPUE for fish >37 cm (grey line with crosses) has dropped since 2009–2010 and fish >45 cm (black line with open squares) have almost disappeared in recent years. Full size image Figure 4: Mean annual catch per unit effort (CPUE) for Eastern Baltic cod. The CPUE for the size group 30–37 cm (black line with triangles) has dramatically increased since the millennium shift, while the CPUE for fish >37 cm (grey line with crosses) has dropped since 2009–2010 and fish >45 cm (black line with open squares) have almost disappeared in recent years. Full size image Changed mortality patterns In addition, comparisons between regularly assessed values of total mortality, Z , by the regional scientific advisor at the International Council for the Exploration of the Sea (ICES) ( www.ices.dk ) and survey-based estimations of Z for fish >37 cm (that is, MLS) showed a deviating pattern over recent years ( Fig. 5 ). Survey-based estimations of Z indicate that mortality for larger fish has remained high, while Z for the length interval 30–37 cm indicates a decline in mortality since the early 2000s; the latter is in agreement with the regular assessment, which includes all fish irrespective of length. 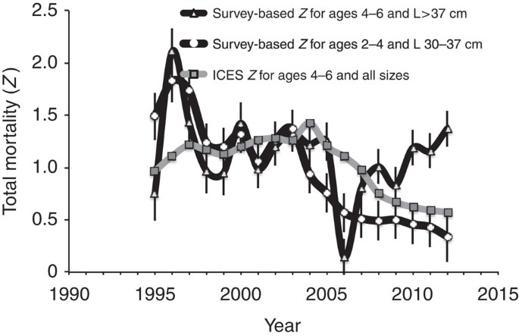Figure 5:Comparison between survey-based estimated total mortality,Z. The total mortality,Z(±s.e., estimated by bootstrapping30), has decreased in recent years for smaller cod (30–37 cm and ages 2–4; black line with open circles) whereasZhas increased for larger cod (>37 cm and ages 4–6; black line with triangles). EstimatedZ, for all sizes and ages 4–6 according to the regular assessment11has been added (grey line with squares) for comparison reasons. Figure 5: Comparison between survey-based estimated total mortality, Z . The total mortality, Z (±s.e., estimated by bootstrapping [30] ), has decreased in recent years for smaller cod (30–37 cm and ages 2–4; black line with open circles) whereas Z has increased for larger cod (>37 cm and ages 4–6; black line with triangles). Estimated Z , for all sizes and ages 4–6 according to the regular assessment [11] has been added (grey line with squares) for comparison reasons. Full size image Accounting for density-dependent effects The decline in L ∞ is correlated to the total number of fish aged ⩾ 2 years in the stock, according to the regular assessment [11] , indicating density dependence ( Fig. 6 ). However, by taking into account changes in selectivity since 1995, modelled natural and fishing mortality rates, and the observed value of L ∞ per year class (see ‘Methods’), we could reconstruct the observed developments in numbers ≤37 and >37 cm, respectively, over time ( Fig. 7a ). By taking into account the observed density dependence of L ∞ , it could be shown that by keeping selectivity low ( L c =30 cm), crowding of fish ≤37 cm can be avoided ( Fig. 7b ). In a simulation, using low and moderately high L ∞ on yield-per-recruit at three levels of fishing mortality for Eastern Baltic cod clearly indicates that variation in selectivity, L c , or fishing mortality, F , is much less important than variation in growth potential L ∞ ( Fig. 8 ). 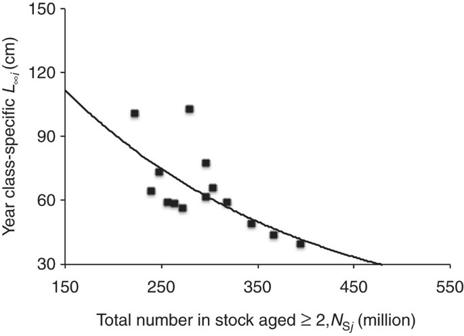Figure 6:Mean asymptotic length in cm,L∞i, for year class,i, as a function of the stock number,Nsj. Nsj, is equivalent to the number of fish at age⩾2 years in million, according to the regular assessment11.Nsjis shifted 2 years forward in the regression for year classes 1995–2008 (L∞i=204.5*e−4.022e−9*Nsj; multipler2=0.54;P<0.001), as to relate the effect ofNsjonL∞iat age 2 years for year-classi. Figure 6: Mean asymptotic length in cm, L ∞ i , for year class, i , as a function of the stock number, N s j . N s j , is equivalent to the number of fish at age ⩾ 2 years in million, according to the regular assessment [11] . N s j is shifted 2 years forward in the regression for year classes 1995–2008 ( L ∞ i =204.5*e −4.022e−9* N s j ; multiple r 2 =0.54; P <0.001), as to relate the effect of N s j on L ∞ i at age 2 years for year-class i . 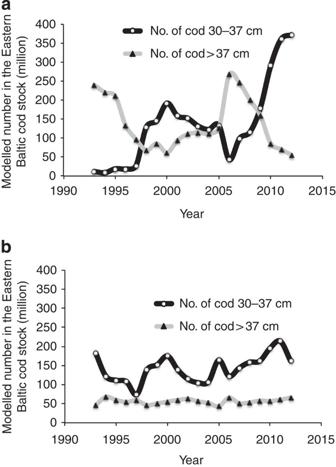Figure 7: Predicted number at length by taking density dependence into account. (a) Predicted numbers of fish at sizes 30–37 (black line and grey circles) and >37 cm (grey line and black triangles) over time from modelled values ofFj,MjandL∞i, and from recruitment values from routine assessment11and imposed changes in selectivity. (b) Number of fish 30–37 (black line and grey circles) and >37 cm (grey line and black triangles) over time, modelled by settingLcat 30 cm,Fjat 0.8 andMjat 0.3, and estimatingL∞iby using the observed density-dependent relationship in Eastern Baltic cod. Full size image Figure 7: Predicted number at length by taking density dependence into account. ( a ) Predicted numbers of fish at sizes 30–37 (black line and grey circles) and >37 cm (grey line and black triangles) over time from modelled values of F j , M j and L ∞ i , and from recruitment values from routine assessment [11] and imposed changes in selectivity. ( b ) Number of fish 30–37 (black line and grey circles) and >37 cm (grey line and black triangles) over time, modelled by setting L c at 30 cm, F j at 0.8 and M j at 0.3, and estimating L ∞ i by using the observed density-dependent relationship in Eastern Baltic cod. 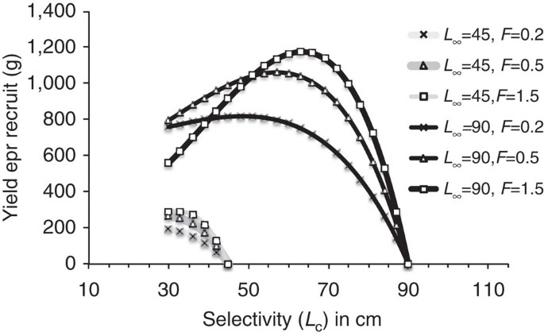Figure 8: Yield per recruit for Eastern Baltic cod at two levels of mean asymptotic length,L∞i. Theoretically estimated yield per recruit,Yw/R, from the Eastern Baltic cod stock at a low (L∞at 45 cm) and high (L∞at 90 cm) productive state as a function of selectivity,Lc, at three levels of fishing mortality (Fat 0.2, 0.5 and 1.5). (L∞at 45/90 cm are shown with grey/black lines, andFat 0.2/0.5/1.5 are shown with crosses/triangles/open squares, respectively). Full size image Figure 8: Yield per recruit for Eastern Baltic cod at two levels of mean asymptotic length, L ∞ i . Theoretically estimated yield per recruit, Y w / R , from the Eastern Baltic cod stock at a low ( L ∞ at 45 cm) and high ( L ∞ at 90 cm) productive state as a function of selectivity, L c , at three levels of fishing mortality ( F at 0.2, 0.5 and 1.5). ( L ∞ at 45/90 cm are shown with grey/black lines, and F at 0.2/0.5/1.5 are shown with crosses/triangles/open squares, respectively). Full size image The lack of cod available to fish in the Eastern Baltic is tightly linked to its lost growth potential, resulting in a steep drop in numbers of fish of fishable size and, furthermore, poor individual status. In fact, L ∞ is at present below or close to L c , which means that few fish are expected to grow above the 50% point of the selectivity ogive, which is equivalent to a fish length of 45 cm. Based on our analysis, the most parsimonious explanation for this process is that increased selectivity has induced a steady increase in number of small-sized fish, which in turn has led to density-dependent growth. The causal mechanism for this process could be related to lower mortality rates for intermediate size groups, partly due to lower catchability as selectivity is increased, and partly due to less predation from larger size groups as they suffer a decline in the relative and absolute abundance over the study period. The process is, then, self-reinforcing: as growth goes down, the number of fish per length group inevitably goes up as long as the recruitment remains at least constant [23] , which seems to be the case [11] . Fishing mortality also appears to be increasing in the size interval still open for exploitation. This implies that a higher fishing effort will not solve the problem. Rather, a combination of both lowered effort and selectivity is required so as to break the present deadlock of density dependence. Lower effort, as being proportionate to F , will also ensure that larger size classes will be re-established, leading to increased natural mortality (M) for smaller size groups due to cannibalism [12] . As we did not model cannibalism effects on mortality, we may have overestimated the fishing effort needed to cull smaller size groups. First, our findings contradict the MSY framework in place [11] . All indicators outside the single-stock assessment results of F msy imply severe economic losses for the fishing industry. In addition, there are apparent risks of fishery-induced evolution in size and age at maturity [24] , not to mention ecosystem losses of eroding important predatory fish from the Baltic Sea ecosystem [13] . Tentatively, given this example, we may conclude that managing with MSY diverts attention from the fact that total allowable catches (TACs) increasingly overshoot biomass availability in Eastern Baltic cod [11] . Meanwhile, the regional advising agency is suggesting a 7% TAC increase for 2014 (ref. 25 ). As a recent higher estimate of F msy allows for even larger increases in TACs, it was noted that even higher exploitation rates will deal with ‘the excessive Eastern cod stock density problem’ [25] and that no regulations of effort will be needed in the future. Second, our results disagree with current policies of increased selectivity [21] . There is still a widespread, and unfortunate, preference for improvements in yield over improvements in CPUE [26] , thereby, ignoring economic constraints as well as the benefits of a more pristine size distribution with higher food web stability [27] . Furthermore, if the lower individual growth potential has indeed been reduced because of factors other than dynamic interplay caused by increased selectivity, lower selectivity is still an appropriate response to the present situation in the Eastern Baltic cod fishery: a reduced number of fish will inevitably increase food resources for the survivors, and thereby restore some of the former growth pattern. The Johannesburg declaration [22] of an ‘MSY target’ for all marine fish stocks was made without reference to the selectivity or effort involved: that is, the costs of fishing, either economic or ecological in nature, were not considered. Instead of a search for a maximum output by fine-tuning selectivity and effort (a solution which will become obsolete as soon as the growth potential of the stock changes), a decrease in effort and selectivity will be a superior risk-averting strategy [16] , [27] , [28] . In fact, it would be much more profitable for individual fishermen to fish slightly less than fishing at MSY ( F msy ), because it would lead to higher CPUE [10] , [16] , and would arguably be more environmentally benign because less effort is involved [26] . Prioritizing robust harvest strategies, where CPUE is a crucial estimate on stock status, is arguably more economical and ecologically safe in the longer perspective compared with options related to yield. Although it was introduced with good intentions, a selectivity shortcut to improve yield, profit and ecosystem structure does not exist. Rather, as is illustrated with this case of the Eastern Baltic cod, the policy of increasing selectivity has altered the ecosystem structure of the Baltic Sea, for which the effect may be augmented in the future if proper actions are not taken. Maps Maps showing the Baltic Sea region and Europe were produced by using the software Ocean Data View ( http://odv.awi.de ). Information on the delineation of ICES subdivisions in the Baltic Sea was gathered at www.ices.dk . Information on commercial landings Data on commercial landings of both western and eastern Baltic cod between 2004 and 2011 were gathered from a fish processing unit in Poland. This data includes information on mean weight, trimming time and fillet yield for fresh fish, collected on a regular basis for all cod processed. Modelling of growth potential Survey age-specific catch rates from ICES survey data for subdivisions 25–29 ( Fig. 1 ) (DATRAS at www.ices.dk ) were used for parameterizing von Bertalanffy’s growth model, as follows [29] : where L i is the expected or average length at time (or age) t , L ∞i is the asymptotic average length of year class i , K is the Brody growth rate coefficient (units are per year) and t 0 is a modelling artefact that represents the time or age when the average length was zero. Modelling of data to the von Bertalanffy growth equation was performed using fisheries stock assessment software (FSA fishR; http://www.rforge.net/FSA/ ). The number of iterations for convergence was set to 50 and different initial values of L ∞i and K were tested so as to let the model converge. L ∞i , which mirrors the feeding conditions of a cohort [16] , was estimated as year class mean for two separate surveys in the first and fourth quarter of the year. Modelling of mortality rates Total mortality, Z j , was determined from survey data using SURBA software [30] . Natural mortality rates, M j , were estimated from life history parameters [31] ( http://cran.r-project.org/web/packages/fishmethods/ ). Modelling of density dependence The relationship between the year class-specific length asymptote, L ∞ i , and stock numbers, in year, j , N s j , was modelled with an exponential function by using modelled values of L ∞ i for year classes 1995–2008 and corresponding summed stock numbers, N s j , in year, j , in million, according to published assessment estimates [11] (see Fig. 6 ) when year class, i , was at age 2 years: Modelling of population dynamics Population numbers of fish ≤37 and >37 cm were modelled by using observed L ∞ i per year class i and by setting growth factor K and reference age t 0 to 0.3 and −0.2, respectively. The mean length, L ij , of year class i at year j was estimated using equation (1). To simulate a normal size distribution at year, j , each year class, i , was divided into seven cohorts, v. Each cohort, v , followed its own growth and population trajectory in the model. Each cohort represents a fixed proportion of the year class, i : 38%, 2 × 15%, 2 × 9.2%, 2 × 6.8%. The corresponding mean length of cohort by year class and year was estimated as L ijv , L ijv ±0.5 s.e. of the mean size, L ijv ±1 SE, L ijv ±1.5 SE. As the mean coefficient of variation of the observed lengths for ages 2–10 years during the time period 1991–2013 was observed at c. 0.2, the mean sizes L ijv of the seven cohorts per year and year class were accordingly estimated as L ijv , L ijv ±0.1 × L ij , L ijv ±0.2 × L ij , L ijv ±0.3 × L i . Number, N , for year class and cohort at year, j , N ivj was determined by the following equation: where N iv ( j −1) is the number of survivors in the preceding year ( j −1) and t is the age interval (set to 1 year). For each year class, i , the starting year of estimation is the year of recruitment at age 2 years, where N iv 2 is the recruitment for year class and cohort at age 2 years, using published assessment recruitment values [11] . Where the mean length of cohort for year class and year was below the 50% point of the selectivity ogive, that is, L ijv < L c , fishing mortality, F j , was set to 0. Modelling of yield To model yields at various levels of exploitation rate E ( E=F / Z ) and selectivity L c , lifetime percentage yield, y , was calculated for L ∞ i at 45 and 90 cm by the following yield function [32] : where Ω n =+1, −3, +3, −1 for n =0, 1, 2 and 3, respectively; c = L c / L ∞ i . Further, m=M/K is a mortality–growth ratio. In this study, M and K were set at 0.3 (that is, m =1). For calculation of yield per recruit Y w / R , the following equation was used as a way to return to original scaling: where Y w is the yield in weight, t r is the age at recruitment to a fishable size and W ∞ i is the mean asymptote weight. W ∞ i was calculated using the weight–length relationship: where published values for Eastern Baltic cod a =0.104 and b =3 were used [9] . How to cite this article: Svedäng, H. & Hornborg, S. Selective fishing induces density-dependent growth. Nat. Commun. 5:4152 doi: 10.1038/ncomms5152 (2014).